TheBrassica oleraceagenome reveals the asymmetrical evolution of polyploid genomes Polyploidization has provided much genetic variation for plant adaptive evolution, but the mechanisms by which the molecular evolution of polyploid genomes establishes genetic architecture underlying species differentiation are unclear. Brassica is an ideal model to increase knowledge of polyploid evolution. Here we describe a draft genome sequence of Brassica oleracea , comparing it with that of its sister species B. rapa to reveal numerous chromosome rearrangements and asymmetrical gene loss in duplicated genomic blocks, asymmetrical amplification of transposable elements, differential gene co-retention for specific pathways and variation in gene expression, including alternative splicing, among a large number of paralogous and orthologous genes. Genes related to the production of anticancer phytochemicals and morphological variations illustrate consequences of genome duplication and gene divergence, imparting biochemical and morphological variation to B. oleracea . This study provides insights into Brassica genome evolution and will underpin research into the many important crops in this genus. B rassica oleracea comprises many important vegetable crops including cauliflower, broccoli, cabbages, Brussels sprouts, kohlrabi and kales. The species demonstrates extreme morphological diversity and crop forms, with various members grown for their leaves, flowers and stems. About 76 million tons of Brassica vegetables were produced in 2010, with a value of 14.85 billion dollars ( http://faostat.fao.org/ ). Most B. oleracea crops are high in protein [1] and carotenoids [2] , and contain diverse glucosinolates (GSLs) that function as unique phytochemicals for plant defence against fungal and bacterial pathogens [3] and on consumption have been shown to have potent anticancer properties [4] , [5] , [6] . B. oleracea is a member of the family Brassicaceae (~\n338 genera and 3,709 species) [7] and one of three diploid Brassica species in the classical triangle of U [8] that also includes diploids B. rapa (AA) and B. nigra (BB) and allotetraploids B. juncea (AABB), B. napus (AACC) and B. carinata (BBCC). These allotetraploid species are important oilseed crops, accounting for 12% of world edible oil production ( http://faostat.fao.org/ ). As the origin and relationship between these species is clear, the timing and nature of the evolutionary events associated with Brassica divergence and speciation can be revealed by interspecific genome comparison. Each of the Brassica genomes retains evidence of recursive whole-genome duplication (WGD) events [9] , [10] ( Supplementary Fig. 1 ) and have undergone a Brassiceae -lineage-specific whole-genome triplication (WGT) [11] , [12] since their divergence from the Arabidopsis lineage. These events were followed by diploidization that involved substantial genome reshuffling and gene losses [11] , [12] , [13] , [14] , [15] . Because of this, Brassica species are a model for the study of polyploid genome evolution ( Supplementary Fig. 2 ), mechanisms of duplicated gene loss, neo- and sub-functionalization, and associated impact on morphological diversity and species differentiation. We report a draft genome sequence of B. oleracea and its comprehensive genomic comparison with the genome of sister species B. rapa , which diverged from a common ancestor ~\n4 MYA. These data provide insights into the dynamics of Brassica genome evolution and divergence, and serve as important resources for Brassica vegetable and oilseed crop breeding. Furthermore, this genome will support studies of the large range of morphological variation found within B. oleracea , which includes sexually compatible crops such as cabbages, cauliflower and broccoli that are important for their economic, nutritional and potent anticancer value. B. oleracea genome assembly and annotation Complementing the sequencing of the smaller B. rapa genome [11] , a draft genome assembly of B. oleracea var. capitata line 02–12 was produced by interleaving Illumina, Roche 454 and Sanger sequence data. This assembly represents 85% of the estimated 630 Mb genome, and includes >98% of the gene space ( Supplementary Methods , Supplementary Tables 1–3, 7 and 8 and Supplementary Fig. 3 ). The assembly was anchored to a new genetic map [16] to produce nine pseudo-chromosomes that account for 72% of the assembly, and validated by comparison with a B. oleracea physical map [17] , a high-density B. napus genetic map [18] and complete BAC sequences ( Supplementary Figs 4–9 and Supplementary Tables 4 and 5 ). For comparative analyses, identical genome annotation pipelines were used for annotation of protein-coding genes and transposable elements (TEs) for B. oleracea and B. rapa . 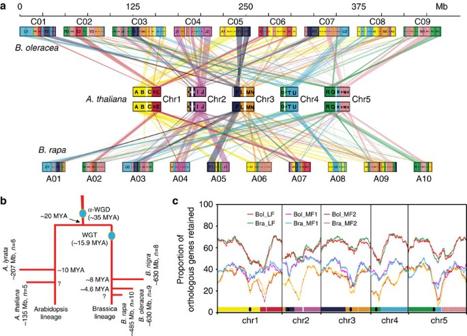Figure 1: Genomic structure and gene retention rates in syntenic regions ofB. oleraceaandB. rapa. (a) Segmental colinearity of the genomes ofB. oleracea,B. rapaandA. thaliana. Syntenic blocks are defined and labelled from A to X (coloured) previously reported inA. thaliana20. (b) Time estimate of WGD and subsequent twoBrassicaspecies divergence. (c) Pattern of retention/loss of orthologous genes on each set of three subgenomic (LF, MF1 and MF2) blocks ofB. oleraceaandB. rapacorresponding toA. thalianaA to X blocks. Thexaxis denotes the physical position of eachA. thalianagene locus. Theyaxis denotes the proportion of orthologous genes retained in theB. oleraceaandB. rapasubgenomic blocks around eachA. thalianagene, where 500 genes flanking each side of a certain gene locus were analysed, giving a total window size of 1,001 genes. A total of 45,758 protein-coding genes were predicted, with a mean transcript length of 1,761 bp, a mean coding length of 1,037 bp, and a mean of 4.55 exons per gene ( Table 1 , Supplementary Methods , Supplementary Table 6 and Supplementary Fig. 10 ), similar to A. thaliana [19] and B. rapa [11] . Publicly available ESTs, together with RNA sequencing (RNA-seq) data generated in this study, support 94% of predicted gene models ( Supplementary Tables 7 and 8 ), and 91.6% of predicted genes have a match in at least one public protein database ( Supplementary Tables 9 and 10 , and Supplementary Fig. 11 ). Of the 45,758 predicted genes, 13,032 produce alternative splicing (AS) variants with intron retention and exon skipping ( Supplementary Table 11 ). Genome annotation also predicted 3,756 non-coding RNAs (miRNA, tRNA, rRNA and snRNA) ( Supplementary Table 12 ). Table 1 Summary of genome assembly and annotation of B. oleracea . Full size table A combination of structure-based analyses and homology-based comparisons resulted in the identification of 13,382 TEs with clearly identified terminal boundaries, including 5,107 retrotransposons and 8,275 DNA transposons ( Supplementary Methods , Supplementary Fig. 12 and Supplementary Table 13 ). These elements together with numerous truncated elements or TE remnants make up 38.80% of the assembled portion of the B. oleracea genome, whereas TEs account for only 21.47% of the B. rapa genome assembly. Copia (11.64%) and gypsy (7.84%) retroelements are the major constituents of the repetitive fraction, and are unevenly distributed across each chromosome, with retrotransposons predominantly found in pericentromeric or heterochromatic regions ( Supplementary Fig. 13 ) in B. oleracea . Tentative physical positions of some of the centromeres were determined based on homologue and phylogenetic analysis of the centromere-specific 76 bp tandem repeats CentBo-1 and CentBo-2 and copia-type retrotransposon (CentCRBo) ( Supplementary Table 14 and Supplementary Figs 14–17 ). The distribution of 45S and 5S rDNA sequences were also visualized by fluorescent in situ hybridization ( Supplementary Figs 18 and 19 ), leading to a predicted karyotype ideogram for B. oleracea ( Supplementary Fig. 20 ). An extra-centromeric locus with colocalized centromeric satellite repeat CentBo-1 and the centromeric retrotransposon CRBo-1 was observed on the long arm of chromosome 6 ( Supplementary Figs 18–20 ). A comprehensive database for the genome information is accessible at http://www.ocri-genomics.org/bolbase/index.html . Conserved syntenic blocks and genome rearrangement after WGT The relatively complete triplicated regions in B. oleracea and B. rapa were constructed and they relate to the 24 ancestral crucifer blocks (A–X) in A. thaliana [20] . Further the triplicated blocks resulting from WGT in the two Brassica species were partitioned into three subgenomes: LF (Least-fractionated), MF1 (Medium-fractionated) and MF2 (Most-fractionated) [11] ( Fig. 1a , Supplementary Methods , Supplementary Tables 15 and 16 , and Supplementary Figs 21–26 ). These syntenic blocks occupy the majority of the genome assemblies of A. thaliana (19,628 genes, 72.24% of 27,169 genes), B. oleracea (26,485 genes, 57.88%) and B. rapa (26,698 genes, 64.84%), and provide a foundation for comparative analyses of chromosomal rearrangement, gene loss and divergence of retained paralogues after WGT. Massive gene loss occurred in an asymmetrical and reciprocal fashion in the three subgenomes of each species and was largely completed before the B. oleracea–B. rapa divergence ( Fig. 1c , Supplementary Tables 17–19 and Supplementary Figs 25–27 ). The timing of this evolutionary process was supported by the estimated timing of WGT ~\n15.9 million years ago (MYA), and species divergence ~\n4.6 MYA, based on synonymous substitution (Ks) rates of genes located in the blocks ( Fig. 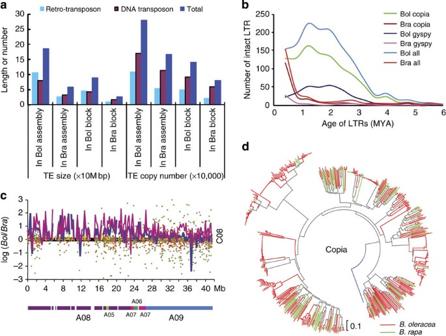Figure 2: TE comparison analyses inB. oleraceaandB. rapa. (a) TE copy number and total length in each assembly andB. oleracea–B. rapasyntenic blocks. (b) The number of intact LTR (Copia-like andGypsy-like) birthed at different times (million years ago, MYA) in the syntenic regions ofB. oleraceaandB. rapa. (c) The comparison of TE distribution and composition inB. oleracea–B. rapasyntenic blocks alongB. oleraceachromosomes. We dividedB. oleracea–B. rapasyntenic region into non-overlapping sliding 200 kb windows to compare TE contents. For each window, the ratio log10(B. oleracea/B. rapa) was calculated for total syntenic block length (blue line), LTR length (purple line), gene length (yellow point), exons length (red point) and intron length (green point). IfB. oleracea>B. rapain absolute length of TE composition in a compared window, the dot or line is above the liney=0. The correspondingB. rapachromosome segments alongB. oleraceaC08 were indicated by coloured bars. All otherB. oleraceachromosomes are showed inSupplementary Fig. 31. (d) Phylogeny of the Copia-like elements as an example of LTR-RTs of the syntenic regions inB. rapaandB. oleracea. The neighbor-joining (NJ) trees were generated based on the conserved RT domain nucleotide sequences using the Kimura two-parameter method68in MEGA4 (ref.69). 1b and Supplementary Table 20 ). Gene loss occurred mainly through small deletions that may be caused by illegitimate recombination [21] , [22] ( Supplementary Fig. 27 ), consistent with observations in other plant genomes. Figure 1: Genomic structure and gene retention rates in syntenic regions of B. oleracea and B. rapa . ( a ) Segmental colinearity of the genomes of B. oleracea , B. rapa and A. thaliana . Syntenic blocks are defined and labelled from A to X (coloured) previously reported in A. thaliana [20] . ( b ) Time estimate of WGD and subsequent two Brassica species divergence. ( c ) Pattern of retention/loss of orthologous genes on each set of three subgenomic (LF, MF1 and MF2) blocks of B. oleracea and B. rapa corresponding to A. thaliana A to X blocks. The x axis denotes the physical position of each A. thaliana gene locus. The y axis denotes the proportion of orthologous genes retained in the B. oleracea and B. rapa subgenomic blocks around each A. thaliana gene, where 500 genes flanking each side of a certain gene locus were analysed, giving a total window size of 1,001 genes. Full size image Abundant genome rearrangement following WGT and subsequent Brassica species divergence resulted in complex mosaics of triplicated ancestral genomic blocks in the A and C genomes ( Fig. 1a and Supplementary Fig. 28 ). At least 19 major, and numerous fine-scale, chromosome rearrangements occurred, which differentiate the two Brassica species ( Supplementary Fig. 29 ). This is in agreement with previous comparative studies based on chromosome painting [12] , [23] and genetic mapping [24] , [25] . The extensive chromosome reshuffling in Brassica is in contrast to that observed in other taxa, such as the highly syntenic tomato–potato and pear–apple genomes, each with longer divergence times and less genome rearrangement [26] , [27] . This difference may be a consequence of mesopolyploidy in Brassica . Greater TEs accumulation in B. oleracea than B. rapa Both retro- (22.13%) and DNA (16.67%) TEs appear to be greater amplified in B. oleracea relative to B. rapa (9.43 and 12.04%) ( Fig. 2a and Supplementary Table 13 ). We constructed 1,362 gap-free contig-contig syntenic regions by clustering orthologous B. rapa — B. oleracea genes using MCscan ( Supplementary Figs 29 and 30 ). The B. oleracea TE length (34.03% of the 259.6M) is 3.4 times greater than that of the syntenic B. rapa regions (16.73% of the 155.0M) ( Fig. 2c , Supplementary Tables 21 and 22 , and Supplementary Fig. 31 ). Phylogenetic analysis revealed that B. oleracea has both more LTR retrotransposon (LTR-RT) families, and more members in most families than B. rapa ( Fig. 2d and Supplementary Figs 12, 32 and 33 ). Furthermore, two new lineages of LTR-RTs, Brassica Copia Retrotransposon and Brassica Gypsy Retrotransposon, were defined in both Brassica species ( Supplementary Fig. 33 ). Analysis of LTR insertion time revealed that ~\n98% of B. oleracea intact LTR-RTs amplified continuously over the ~\n4 million years (MY) since the B. oleracea – B. rapa split, whereas ~\n68% of B. rapa intact LTR-RTs amplified rapidly within the last 1 MY, predominantly in the recent 0.2 MY ( Fig. 2b and Supplementary Fig. 34 ). Hence, LTR-RTs expanded more in the intergenic space of euchromatic regions in B. oleracea than B. rapa . This agrees with previous observations based on comparison of BAC sequences between the A and C genomes [28] . As a consequence of continuous TE amplification over the last 4 MY, the genome size of B. oleracea is ~\n30% larger than that of B. rapa although the two genomes share the same ploidy and are largely collinear. Figure 2: TE comparison analyses in B. oleracea and B. rapa. ( a ) TE copy number and total length in each assembly and B. oleracea–B. rapa syntenic blocks. ( b ) The number of intact LTR ( Copia -like and Gypsy -like) birthed at different times (million years ago, MYA) in the syntenic regions of B. oleracea and B. rapa . ( c ) The comparison of TE distribution and composition in B. oleracea–B. rapa syntenic blocks along B. oleracea chromosomes. We divided B. oleracea–B. rapa syntenic region into non-overlapping sliding 200 kb windows to compare TE contents. For each window, the ratio log 10 ( B. oleracea/B. rapa ) was calculated for total syntenic block length (blue line), LTR length (purple line), gene length (yellow point), exons length (red point) and intron length (green point). If B. oleracea > B. rapa in absolute length of TE composition in a compared window, the dot or line is above the line y =0. The corresponding B. rapa chromosome segments along B. oleracea C08 were indicated by coloured bars. All other B. oleracea chromosomes are showed in Supplementary Fig. 31 . ( d ) Phylogeny of the Copia-like elements as an example of LTR-RTs of the syntenic regions in B. rapa and B. oleracea . The neighbor-joining ( NJ ) trees were generated based on the conserved RT domain nucleotide sequences using the Kimura two-parameter method [68] in MEGA4 (ref. 69 ). Full size image Species-specific genes and tandemly duplicated genes While the genomes of B. oleracea and B. rapa are highly similar in terms of total gene clusters/sequences and the gene number in each cluster, there are also a large number of species-specific genes in the two species. A total of 66.5% (34,237 genes) of B. oleracea genes and 74.9% (34,324) of B. rapa genes were clustered into OrthoMCL groups ( Supplementary Table 23 and Supplementary Fig. 35 ). We identified 9,832 B. oleracea -specific and 5,735 B. rapa -specific genes, of which 77% were supported by gene expression and/or a clear Arabidopsis homologue ( Supplementary Table 24 ). Of them, >90% of these specific genes were validated for their absence in the counterpart genomes by reciprocal mapping of raw clean reads ( Supplementary Tables 25 and 26 ). Most Brassica -specific genes are randomly distributed along the chromosomes ( Supplementary Figs 36 and 37 ). More than 80% of the species-specific genes were surrounded by non-specific genes ( Supplementary Fig. 38 ), suggesting that deletion of individual genes may be the major mechanism underlying gene loss and the difference in gene numbers between B. oleracea and B. rapa . Tandem duplication produces clusters of duplicated genes and contributes to the expansion of gene families [29] . We identified 1,825, 2,111 and 1,554 gene clusters containing 4,365, 5,181 and 4,170 tandemly duplicated genes in B. oleracea , B. rapa and A. thaliana , respectively ( Fig. 3a , Supplementary Tables 27 and 28 and Supplementary Fig. 39 ). The wide range of sequence divergence of tandem gene pairs in each species suggests that tandem gene duplication occurred continuously throughout the evolutionary history of these species, rather than in discrete bursts ( Supplementary Figs 40 and 41 ). Their continuous and asymmetrical occurrence after species divergence resulted in 522, 697 and 815 species-specific tandem clusters in the three genomes. The frequency of tandem duplication is independent of the total gene content, suggesting that genome triplication has not inhibited its occurrence. Tandemly duplicated genes are preferentially enriched for gene ontology (GO) categories related to defence response and pathways related to secondary metabolism such as indole alkaloid biosynthesis and tropane, piperidine and pyridine alkaloid biosynthesis ( Fig. 3b , Supplementary Tables 29–32 and Supplementary Fig. 42 ). 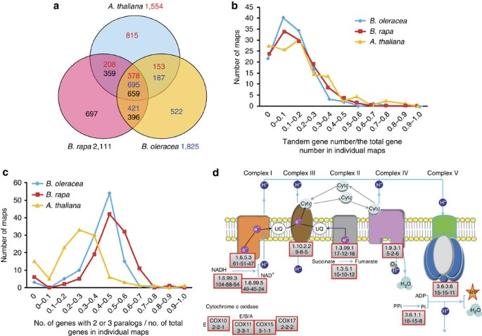Figure 3: The duplicated genes derived from tandem duplication and whole-genome duplications inBrassicagenomes. (a) A Venn diagram showing shared and specific tandem duplication events inA. thaliana,B. rapaandB. oleracea. (b,c) Distribution of tandem genes and WGT/WGD-derived paralogues in the KEGG pathway maps inB. oleracea(bol),B. rapa(bra) andA. thaliana(ath). For each KEGG pathway map, the proportion of the number of duplicated genes or paralogues to the total genes was calculated (xaxis) and the number of maps whose tandem gene proportion fell in a range was shown on theyaxis. (d) Oxidative phosphorylation pathway enriched by WGT-derived paralogous genes in theBrassicagenomes. The gene copy number for each KO enzyme inB. oleracea,B. rapaandA. thalianawere shown (dash-connected) under the KO enzyme number. Over 44.0 and 51.9% of the NBS-encoding resistance genes are tandemly duplicated in B. oleracea and B. rapa , respectively ( Supplementary Table 33 ). Figure 3: The duplicated genes derived from tandem duplication and whole-genome duplications in Brassica genomes. ( a ) A Venn diagram showing shared and specific tandem duplication events in A. thaliana , B. rapa and B. oleracea . ( b , c ) Distribution of tandem genes and WGT/WGD-derived paralogues in the KEGG pathway maps in B. oleracea (bol), B. rapa (bra) and A. thaliana (ath). For each KEGG pathway map, the proportion of the number of duplicated genes or paralogues to the total genes was calculated ( x axis) and the number of maps whose tandem gene proportion fell in a range was shown on the y axis. ( d ) Oxidative phosphorylation pathway enriched by WGT-derived paralogous genes in the Brassica genomes. The gene copy number for each KO enzyme in B. oleracea , B. rapa and A. thaliana were shown (dash-connected) under the KO enzyme number. Full size image Biased loss and retention of genes after WGT/WGD Following polyploidization, reversion of gene numbers towards diploid levels through gene loss has been widely observed in plants [30] . However, in Brassica this only appears to be true for collinear genes in the conserved syntenic regions, with a loss of ~\n60% of the predicted post-triplication gene set, nearly restoring the pre-triplication gene number. This is reflected in an overall retention rate of 1.2-fold of A. thaliana orthologous genes in corresponding syntenic regions ( Fig. 1c and Supplementary Table 18 ). In contrast, in terms of genes that have no collinear gene in A. thaliana and either Brassica species (hereafter called non-collinear genes), gene retention rates is 2.5-fold the A. thaliana gene number in B. oleracea and 1.9-fold in B. rapa , both significantly higher than the expected rates ( P value <2.2e–16; Supplementary Table 34 ). For these retained genes, the numbers of the genes that are common in the two Brassica species are 11,746 in B. oleracea and 10,411 in B. rapa . Most of these genes are supported by expression and/or the presence of an Arabidopsis homologue ( Supplementary Table 35 ). More than 61% of these genes have homologues present as collinear genes and 16% also are homologous to other non-collinear genes, indicating gene movement from triplicated syntenic regions and being similar to observations in A. thaliana , where half of the genes are nonsyntenic within rosids [31] . This suggests that the breakdown of the triplicated syntenic relationship has not only prevented gene loss and a move towards pre-triplication gene numbers but has also maintained a higher gene density, and thus maintained WGT-derived genes for species evolution. The presence of a large number of the retained paralogous genes in the syntenic regions led us to examine whether genes in some functional categories have preferentially been over-retained, as observed in other plants [29] . The results indicate that WGT-produced paralogous genes are over-retained in GO categories associated with regulation of metabolic and biosynthetic processes, RNA metabolism and transcription factors ( Supplementary Table 36 and Supplementary Figs 43–45 ), and the two Brassica species exhibit similar patterns of gene category retention. From a study of KEGG pathways, we also found that WGT-produced Brassica paralogous genes contribute 40–60% of total genes for 90% of KEGG pathways ( Fig. 3c and Supplementary Fig. 43 ), and are functionally enriched in primary or core metabolic processes such as oxidative phosphorylation, carbon fixation, photosynthesis, circadian rhythm [32] and lipid metabolism ( Supplementary Tables 36 and 37 and Supplementary Figs 43–45 ). Notably, the pathways associated with energy metabolism have been enhanced in both Brassica species. For instance, in the oxidative phosphorylation pathway, there are 161 genes in A. thaliana , but 241 in B. oleracea and 208 in B. rapa . The majority (143/241 and 142/208) of these Brassica genes are multiple paralogues residing in the triplicated syntenic regions, and more than half of these paralogues have been retained as three copies, significantly higher than observed for other genes in the triplication regions ( Fig. 3d and Supplementary Fig. 43 ). Phylogenetic analyses show that WGT led to an expansion of genes involved in auxin functioning (AUX, IAA, GH3, PIN, SAUR, TAA, TIR, TPL and YUCCA), morphology specification (TCP), and flowering time control (FLC, CO, VRN1, LFY, AP1 and GI) ( Supplementary Table 38 and Supplementary Figs 46–61 ), and that most Arabidopsis genes in these families have two or three orthologs in Brassica species. These WGT-produced duplicated genes may provide important sources of evolutionary innovation [33] and contribute to the extreme morphological diversity in Brassica species. Divergence of duplicated genes in the Brassica genomes The largest genetic foundation for plant genome evolution and new species formation is the differentiation of retained paralogous and orthologous genes. Around 38% (4,302/11,493) of all paralogous gene pairs in B. oleracea and ~\n36% (4,089/11,448) in B. rapa have different predicted exon numbers ( Supplementary Data 1 , Supplementary Tables 39 and 40 and Supplementary Fig. 62 ). There are 6,571 orthologous gene pairs with different exon numbers, accounting for 27.6% of total gene pairs (23,823). Some paralogous or orthologous pairs have high Ks values and low sequence similarity ( Supplementary Fig. 63 ), indicating sequence differentiation. Of these paralogous genes, some offer appreciable opportunity for non-reciprocal DNA exchanges (gene conversion). About 8% of the 4,296 homologous quartets in B. rapa and B. oleracea have been affected by gene conversion ( Fig. 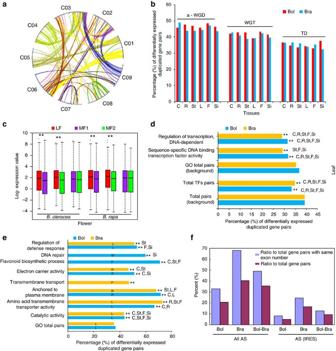Figure 4: Divergence ofBrassicaparalogous and orthologous genes inB. oleraceaandB. rapa. (a) Genome-wide gene conversion inB. oleracea. The conversion inB. rapais showed inSupplementary Fig. 64. (b) The ratio of differentially expressed duplicated gene pairs derived from different duplications: alpha whole-genome duplication (α-WGD),Brassiceae-lineage WGT, tandem duplication (TD). Bol,B. oleracea; Bra,B. rapa. C: callus; R: root; St: stem; L: leaf; F: flower; Si: silique. The differentially expressed duplicated gene pairs were defined as fold change >2 and false discovery rate (FDR) <0.05 or gene pair where expression was detected for only one gene within gene pairs (FDR <0.05). (c) Box and whisker plots for differentiated expression for three subgenomes (LF, MF1 and MF2) in flower tissue ofB. oleraceaandB. rapa. For the other tissues, seeSupplementary Fig. 67. (d) The duplicated gene pairs belonging to transcription factors (TFs) and its related GO terms contain a significantly lower ratio of differentially expressed duplicated gene pairs than the average at the genome-wide level in leaf (values given) and other tissues (values not presented) (Supplementary Table 45). (e) The GO terms (left) in which the duplicated gene pairs contain a significantly higher ratio of differentially expressed duplicated gene pairs than the average ratio at the genome-wide level in leaf and other tissues (Supplementary Table 46). Values from one tissue were presented and the other tissues were indicated with abbreviated letters to the right if expression in these tissues is significantly higher. (f) Expression variation caused by divergence (either different variants or differential expression of the same variants) of alternative splicing (AS) variants in WGT paralogous gene pairs with identical numbers of exons and in Bol–Bra orthologous gene pairs. IRES denotes types of intron retention and exon skipping. 4a , Supplementary Table 41 and Supplementary Fig. 64 ) and about one-sixth (53) of converted genes were inferred to have experienced independent conversion events in both Brassica species, a parallelism sometimes observed in other plants [11] , [34] . Around 40–44% of conversion events involved paralogues in the less-fractionated subgenomes LF in both species, substantially higher than the other two subgenomes ( Supplementary Table 41 ). This finding suggests that gene conversion is related to homologous gene density, which determines the likelihood of illegitimate recombination. Figure 4: Divergence of Brassica paralogous and orthologous genes in B. oleracea and B. rapa . ( a ) Genome-wide gene conversion in B. oleracea . The conversion in B. rapa is showed in Supplementary Fig. 64 . ( b ) The ratio of differentially expressed duplicated gene pairs derived from different duplications: alpha whole-genome duplication (α-WGD), Brassiceae -lineage WGT, tandem duplication (TD). Bol, B. oleracea ; Bra, B. rapa . C: callus; R: root; St: stem; L: leaf; F: flower; Si: silique. The differentially expressed duplicated gene pairs were defined as fold change >2 and false discovery rate (FDR) <0.05 or gene pair where expression was detected for only one gene within gene pairs (FDR <0.05). ( c ) Box and whisker plots for differentiated expression for three subgenomes (LF, MF1 and MF2) in flower tissue of B. oleracea and B. rapa . For the other tissues, see Supplementary Fig. 67 . ( d ) The duplicated gene pairs belonging to transcription factors (TFs) and its related GO terms contain a significantly lower ratio of differentially expressed duplicated gene pairs than the average at the genome-wide level in leaf (values given) and other tissues (values not presented) ( Supplementary Table 45 ). ( e ) The GO terms (left) in which the duplicated gene pairs contain a significantly higher ratio of differentially expressed duplicated gene pairs than the average ratio at the genome-wide level in leaf and other tissues ( Supplementary Table 46 ). Values from one tissue were presented and the other tissues were indicated with abbreviated letters to the right if expression in these tissues is significantly higher. ( f ) Expression variation caused by divergence (either different variants or differential expression of the same variants) of alternative splicing (AS) variants in WGT paralogous gene pairs with identical numbers of exons and in Bol–Bra orthologous gene pairs. IRES denotes types of intron retention and exon skipping. Full size image Analysis of RNA-seq data generated from callus, root, leaf, stem, flower and silique of B. oleracea and B. rapa suggests that >40% of WGT paralogous gene pairs are differentially expressed in these species ( Fig. 4b and Supplementary Fig. 65 ), suggesting potential subfunctionalization of these genes. In both species, a general trend of expression differentiation was alpha-WGD paralogous genes (~\n46%) > WGT paralogous genes (~\n42%) > tandemly duplicated genes (~\n35%) ( Fig. 4b , Supplementary Fig. 66 and Supplementary Tables 42 and 43 ). Different tissues harbour approximately the same number of differentially expressed duplicates, but this number was slightly higher in flower tissue. The expression level of genes in the LF subgenome was significantly higher than corresponding syntenic genes in the more fractionated subgenomes (MF1 and MF2) while no expression dominance relationship was observed between the subgenomes MF1 and MF2 ( Fig. 4c , Supplementary Table 44 and Supplementary Fig. 67 ). Duplicated transcription factor gene pairs showed less differentiated expression (~\n38%) than the expected ratio at the genome-wide level ( Fig. 4d and Supplementary Table 45 ), while paralogues with GO categories related to membrane, catalytic activity and defence response exhibited a higher ratio of differentiated expression ( Fig. 4e and Supplementary Table 46 ). Of B. oleracea–B. rapa orthologous gene pairs (23,823 in total), ~\n42% were differentially expressed across all tissues ( Supplementary Tables 42 and 43 ). Furthermore, many paralogues generate different transcripts, resulting in expression differentiation. Analysis of AS variants of paralogous gene pairs that have identical numbers of exons demonstrated that these variants (either different variants or differential expression of the same variants) cause >20% and >44% of such paralogous genes to be differentially expressed in B. oleracea and B. rapa , respectively ( Fig. 4f and Supplementary Table 47 ). For orthologous gene pairs of B. oleracea and B. rapa , 35.5% (8,467) of gene pairs showed differential expression due to AS variation. When only counting intron retention and exon skipping, 9.3% (2,215) of gene pairs differ. Divergence in AS variants of gene pairs presents an important layer of gene regulation, as reported [35] , [36] , [37] , [38] , and thus provides a genetic basis for species evolution and new species formation. Unique GSLs metabolism pathways GSLs and hydrolysis products have been of long-standing interest due to their role in plant defence and anticancer properties. Compared with B. rapa and B. napus , B. oleracea has the greatest GSL profile diversity, with wide qualitative and quantitative variation [39] , [40] . We identified 101 and 105 GSL biosynthesis genes in B. rapa and B. oleracea , respectively, and 22 GSL catabolism genes in each species ( Fig. 5a , Supplementary Table 48 and Supplementary Data 2 ). In the GSL biosynthesis and catabolism pathways, tandem genes (41.4%, 40.7% and 33.9% in A. thaliana , B. oleracea and B. rapa , respectively) were present in a much higher proportion than the genome-wide average ( Supplementary Table 32 ). The observed variation of GSL profiles is mainly attributed to the duplication of two genes, methylthioalkylmalate ( MAM ) synthase and 2-oxoglutarate-dependent dioxygenase ( AOP ). 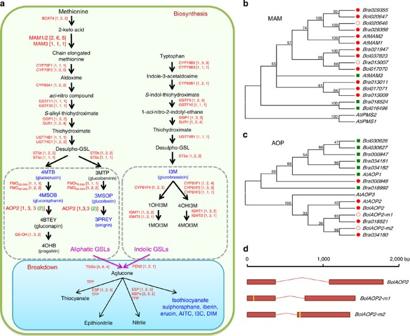Figure 5: Whole-genome-wide comparison of genes involved in glucosinolate metabolism pathways inB. oleraceaand its relatives. (a) Aliphatic and indolic GSL biosynthesis and catabolism pathways inA. thaliana,B. oleraceaandB. rapa. The copy number of GSL biosynthetic genes inA. thaliana,B. rapaandB. oleraceaare listed in square brackets, respectively. Potential anticancer substances/precursors are highlighted in blue bold. Two important amino acid chain elongation and side-chain modification lociMAMsandAOP2are highlighted in red bold, within the number in the green bracket representing the number of non-functional genes. (b,c) The neighbour-joining (NJ) trees of MAM and AOP genes were generated based on the aligned coding sequences and 100 bootstrap repeats. The silenced genes are indicated by red hollow circle, expressed functional genes are represented by red solid disc and green rectangle. InA. thalianaecotype Columbia there are just MAM1 and MAM3. (d) ThreeB. oleracea AOP2loci among which are one functionalAOP2and two mutatedAOP2. 1MOI3M: 1-methoxyindol-3-ylmethyl GSL; 1OHI3M: 1-hydroxyindol-3-ylmethyl GSL; 3MSOP: 3-methylsulfinylpropyl GSL; 3MTP: 3-methylthiopropyl GSL; 3PREY: 2-Propenyl GSL; 4BTEY: 3-butenyl GSL; 4MOI3M: 4-methoxyindol-3-ylmethyl GSL; 4OHB, 4-hydroxybutyl GSL; 4OHI3M: 4-hydroxyindol-3-ylmethyl GSL; 4MSOB: 4-methylsulfinylbutyl GSL; 4MTB, 4-methylthiobutyl GSL; AITC: allyl isothiocyanate; I3C: indole-3-carbinol; I3M: indolyl-3-methyl GSL; DIM: 3,3′-diindolymethane; MAM: methylthioalkylmalate; AOP: 2-oxoglutarate-dependent dioxygenase. Figure 5: Whole-genome-wide comparison of genes involved in glucosinolate metabolism pathways in B. oleracea and its relatives. ( a ) Aliphatic and indolic GSL biosynthesis and catabolism pathways in A. thaliana , B. oleracea and B. rapa . The copy number of GSL biosynthetic genes in A. thaliana , B. rapa and B. oleracea are listed in square brackets, respectively. Potential anticancer substances/precursors are highlighted in blue bold. Two important amino acid chain elongation and side-chain modification loci MAMs and AOP2 are highlighted in red bold, within the number in the green bracket representing the number of non-functional genes. ( b , c ) The neighbour-joining (NJ) trees of MAM and AOP genes were generated based on the aligned coding sequences and 100 bootstrap repeats. The silenced genes are indicated by red hollow circle, expressed functional genes are represented by red solid disc and green rectangle. In A. thaliana ecotype Columbia there are just MAM1 and MAM3. ( d ) Three B. oleracea AOP2 loci among which are one functional AOP2 and two mutated AOP2 . 1MOI3M: 1-methoxyindol-3-ylmethyl GSL; 1OHI3M: 1-hydroxyindol-3-ylmethyl GSL; 3MSOP: 3-methylsulfinylpropyl GSL; 3MTP: 3-methylthiopropyl GSL; 3PREY: 2-Propenyl GSL; 4BTEY: 3-butenyl GSL; 4MOI3M: 4-methoxyindol-3-ylmethyl GSL; 4OHB, 4-hydroxybutyl GSL; 4OHI3M: 4-hydroxyindol-3-ylmethyl GSL; 4MSOB: 4-methylsulfinylbutyl GSL; 4MTB, 4-methylthiobutyl GSL; AITC: allyl isothiocyanate; I3C: indole-3-carbinol; I3M: indolyl-3-methyl GSL; DIM: 3,3′-diindolymethane; MAM: methylthioalkylmalate; AOP: 2-oxoglutarate-dependent dioxygenase. Full size image In Arabidopsis , the MAM family contains three tandemly duplicated and functionally diverse members ( MAM1 , MAM2 and MAM3 ), and functional analysis demonstrated that MAM2 (absent in ecotype Columbia) and MAM1 catalyses the condensation reaction of the first and the first two elongation cycles for the synthesis of dominant 3 and 4 carbon (C) side-chain aliphatic GSLs, respectively [40] , [41] , while MAM3 is assumed to contribute to the production of all GSL chain lengths [42] . In B. rapa and B. oleracea , MAM1 / MAM2 genes experienced independent tandem duplication to produce 6 and 5 orthologs respectively ( Fig. 5b,c ). The main GSLs in B. oleracea are 4C and 3C GSLs (progoitrin, gluconapin, glucoraphanin and sinigrin) [43] , while those in B. rapa are 4C and 5C GSLs (gluconapin and glucobrassicanapin) [39] ( Fig. 5a ). Based on the results of expression and phylogenetic analyses, we found a pair of genes Bol017070 and Bra013007, which are the only orthologous genes showing high expression in B. oleracea but silenced in B. rapa ( Fig. 5a ). This expression difference most likely leads to greater accumulation of the 3C GSL anticancer precursor sinigrin in B. oleracea . Meanwhile, the expression level of MAM3 in B. rapa is much higher than in B. oleracea , explaining the accumulation of 5C GSL glucobrassicanapin in B. rapa . Other genes affecting specific anticancer GLS products are AOPs. Previously, research has reported four gene loci involved in the side-chain modifications of aliphatic GSLs in Arabidopsis . Two tandemly duplicated genes AOP2 and AOP3 catalyse the formation of alkenyl and hydroxyalkyl GSLs, respectively. When both AOPs are non-functional, the plant accumulates the precursor methylsulfinyl alkyl GSL. We identified three AOP2 genes in B. oleracea ( Fig. 5d ), but two are non-functional due to the presence of premature stop codons. In contrast, all three AOP2 copies are functional in B. rapa [44] . No AOP3 homologue has been identified in Brassica . This analysis supports GSL content surveys and explains why glucoraphanin is abundant in B. oleracea , but not in B. rapa . The Brassica genomes experienced WGT [11] , [12] , [25] followed by massive gene loss and frequent reshuffling of triplicated genomic blocks. Analysis of retained or lost genes following triplication identified over-retention of genes for metabolic pathways such as oxidative phosphorylation, carbon fixation, photosynthesis and circadian rhythm [32] , which may contribute to polyploid vigour [45] . Fewer lost genes were observed in the less-fractionated subgenome, possibly due to expression dominance as reported in maize [46] . Gene expression analysis revealed extensive divergence and AS variants between duplicate genes. This subfunctionalization or neofunctionalization of duplicated genes provides genetic novelty and a basis for species evolution and new species formation. For example, TF genes that are considered to be conserved still have more than 38% of paralogous pairs showing differential expression across tissues although this percentage is lower than the average from all duplicated genes. Gene expression variation may contribute to an increased complexity of regulatory networks after polyploidization. The multi-layered asymmetrical evolution of the Brassica genomes revealed in this study suggests mechanisms of polyploid genome evolution underlying speciation. Asymmetrical gene loss between the Brassica subgenomes, the asymmetrical amplification of TEs and tandem duplications, preferential enrichment of genes for certain pathways or functional categories, and divergence in DNA sequence and expression, including alternative splicing among a large number of paralogous and orthologous genes, together shape a route for genome evolution after polyploidization. A molecular model of polyploid genome evolution through these asymmetrical mechanisms is summarized in Supplementary Fig. 2 . The additional information of accessible large datasets and resource was provided in Supplementary Table 49 . In summary, the B. oleracea genomic sequence, its features in comparison with its relatives, and the genome evolution mechanisms revealed, provide a fundamental resource for the genetic improvement of important traits, including components of GSLs for anticancer pharmaceuticals. The genome sequence has also laid a foundation for investigation of the tremendous range of morphological variation in B. oleracea as well as supporting genome analysis of the important allotetraploid crop B. napus (canola or rapeseed). Sample preparation and genome sequencing A B. oleracea sp. capitata homozygous line 02–12 with elite agronomic characters and widely used as a parent in hybrid breeding was used for the reference genome sequencing ( Supplementary Methods ). The seedlings of plants were collected and genomic DNA was extracted from leaves with a standard CTAB extraction method. Illumina Genome Analyser whole-genome shotgun sequencing combined with GS FLX Titanium sequencing technology was used to achieve a B. oleracea draft genome. We constructed a total of 35 paired-end sequencing libraries with insertion sizes of 180 base pairs (bp), 200 bp, 350 bp, 500 bp, 650 bp, 800 bp, 2 kb, 5 kb, 10 kb and 20 kb following a standard protocol provided by Illumina ( Supplementary Methods ). Sequencing was performed using Illumina Genome Analyser II according to the manufacturer’s standard protocol. Genome assembly and validation We took a series of checking and filtering measures on reads following the Illumina-Pipeline, and low-quality reads, adaptor sequences and duplicates were removed ( Supplementary Methods ). The reads after the above filtering and correction steps were used to perform assembly including contig construction, scaffold construction and gap filling using SOAPdenovo1.04 ( http://soap.genomics.org.cn/ ) ( Supplementary Methods ). Finally, we used 20-kb-span paired-end data generated from the 454 platform and 105-kb-span BAC-end data downloaded from NCBI ( http://www.ncbi.nlm.nih.gov/nucgss?term=BOT01 ) to extend scaffold length ( Supplementary Methods ). The B. oleracea genome size was estimated using the distribution curve of 17-mer frequency ( Supplementary Methods ). To anchor the assembled scaffolds onto pseudo-chromosomes, we developed a genetic map using a double haploid population with 165 lines derived from a F1 cross between two homozygous lines 02–12 (sequenced) and 0188 (re-sequenced). The genetic map contains 1,227 simple sequence repeat markers and single nucleotide polymorphism markers in nine linkage groups, which span a total of 1,180.2 cM with an average of 0.96 cM between the adjacent loci [16] . To position these markers to the scaffolds, marker primers were compared with the scaffold sequences using e-PCR (parameters -n2 -g1 –d 400–800), with the best-scoring match chosen in case of multiple matches. We validated the B. oleracea genome assembly by comparing it with the published physical map constructed using 73,728 BAC clones ( http://lulu.pgml.uga.edu/fpc/WebAGCoL/brassica/WebFPC/ ) [17] and a genetic map from B. napus [18] ( Supplementary Methods ). Eleven Sanger-sequenced B. oleracea BAC sequences were used to assess the assembled genome using MUMmer-3.22 ( http://mummer.sourceforge.net/ ) ( Supplementary Methods ). Gene prediction and annotation Gene prediction was performed on the genome sequence after pre-masking for TEs ( Supplementary Methods ). Gene prediction was processed with the following steps: (i) De novo gene prediction used AUGUSTUS [47] and GlimmerHMM [48] with parameters trained from A. thaliana genes. (ii) For homologue prediction, we mapped the protein sequences from A. thaliana , O. sativa , C. papaya , V. vinifera and P. trichocarpa to the B. oleracea genome using tblastn with an E -value cutoff of 10 −5 , and used GeneWise (Version 2.2.0) [49] for gene annotation. (iii) For EST-aided annotation, the Brassica ESTs from NCBI were aligned to the B. oleracea genome using BLAT (identity ⩾ 0.95, coverage ⩾ 0.90) and further assembled using PASA [50] . Finally, all the predictions were combined using GLEAN [51] to produce the consensus gene sets. Functional annotation of B. oleracea genes was based on comparison with SwissProt, TrEMBL, Interproscan and KEGG proteins databases. The tRNA genes were identified by tRNAscan-SE using default parameters [52] . Then rRNAs were compared with the genome using blastn. Other non-coding RNAs, including miRNA, snRNA, were identified using INFERNAL [53] by comparison with the Rfam database. TE annotation LTR-RTs were initially identified using the LTR_STRUC [54] programme, and then manually annotated and checked based on structure characteristics and sequence homology. Refined intact elements were then used to identify other intact elements and solo LTRs [55] . All the LTR-RTs with clear boundaries and insertion sites were classified into superfamilies ( Copia -like, Gypsy -like and Unclassified retroelements) and families relying on the internal protein sequence, 5′, 3′ LTRs, primer-binding site and polypurine tracts. Non-LTR-RTs (Long interspersed nuclear element, LINE and Short interspersed nuclear element, SINE) and DNA transposons ( Tc1-Mariner , hAT , Mutator , Pong , PIF-Harbinger , CACTA and miniature inverted repeat TE) were identified using conserved protein domains of reverse transposase or transposase as queries to search against the assembled genome using tblastn. Further upstream and downstream sequences of the candidate matches were compared with each other to define their boundaries and structure [56] . Helitron elements were identified by the HelSearch 1.0 programme [57] and manually inspected. All the TE categories were identified according to the criteria described previously [58] . Typical elements of each category were selected and mixed together as a database for RepeatMasker [59] analysis. Around 20 × coverage of shotgun reads randomly sampled from the two Brassica genomes were masked by the same TE data set to confirm the different accumulation of TEs between the two genomes. Syntenic block construction of B. oleracea and its relatives We used the same strategy as described in the B. rapa genome paper [11] to construct syntenic blocks between species ( Supplementary Methods ). The all-against-all blastp comparison ( E -value ≤ 1e–5) provided the gene pairs for syntenic clustering determined by MCScan (MATCH_SCORE: 50, MATCH_SIZE: 5, GAP_SCORE: –3, E_VALUE: 1E–05). As applied in B. rapa [11] , we assigned and partitioned multiple B. oleracea or B. rapa chromosomal segments that matched the same A. thaliana segment (‘A to X’ numbering system in A. thaliana [22] ) into three subgenomes: LF, MF1 and MF2. OrthoMCL clustering To identify and estimate the number of potential orthologous gene families between B. oleracea , B. rapa , A. thaliana , C. papaya , P. trichocarpa , V. vinifera , S. bicolor and O. sativa , and also between B. oleracea and B. rapa , we applied the OrthoMCL pipeline [60] using standard settings (blastp E value <1 × 10 −5 and inflation factor =1.5) to compute the all-against-all similarities. Phylogenetic analysis of gene families We performed comparative analysis of trait-related gene families. Genes from grape, papaya and Arabidopsis were downloaded from the GenoScope database ( http://www.genoscope.cns.fr/externe/GenomeBrowser/Vitis/ ), the Hawaii Papaya Genome Project ( http://asgpb.mhpcc.hawaii.edu/papaya/ ), and the Arabidopsis Information Resource ( http://www.arabidopsis.org/ ). Previously reported Arabidopsis and Brassica gene sequences were downloaded from TAIR ( http://www.arabidopsis.org/ ) and BRAD ( http://brassicadb.org/brad/ ). The protein sequences of the genes were used to determine homologues in grape, papaya, Arabidopsis , B. oleracea and B. rapa by performing blast comparisons with an E -value 1e–10. The Clustal [61] programs were used for multiple sequence alignment. Alignment of the small family of GI genes was performed using MEGA5 [62] to conduct neighbour-joining analysis with default parameters and subjected to careful manual checks to remove highly divergent sequences from further analysis. While for other genes, often found in families of tens of genes, the phylogenetic analysis were performed by PhyML [63] , which can accommodate quite divergent sequences by implementing a maximal likelihood approach with initial analysis based on neighbour-joining method. During these analyses, we constructed trees using both CDS and protein sequence, and the protein-derived tree was used to show the phylogeny if not much incongruity was found. Bootstrapping was performed using 100 repetitive samplings for each gene family. All the inferred trees were displayed using MEGA5 (ref. 62 ). The multiple sequence alignment of these families was provided as Supplementary Data 3 . Differential expression of duplicated genes across tissues RNA-seq reads were mapped to their respective locations on the reference genome using Tophat [64] . Uniquely aligned read counts were calculated for each gene for each tissue sample. We performed the exact conditional test of two Poisson rates on read counts of duplicated genes to test the differential expression of duplicated genes, according to the method applied in soybean [65] , [66] . For each duplicated gene pair (for example, genes A and B), read counts and gene length were denoted as Ea and La for gene A, and Eb and Lb for gene B, respectively. The read counts of the genes A and B were assumed to follow the Poisson distributions with rates λA =Ra × La and λB =Rb × Lb. Under the null hypothesis of equal expression of the genes A and B, that is, Ra=Rb, the conditional distribution of Ea given Ea+Eb= k follows a binomial distribution with success probability P =λa/(λa+λb)=La/(La+Lb). The P values were computed and further adjusted to maintain the false discovery rate at 0.05 across gene pairs using the Benjamini–Hochberg method [67] . Statistical analysis The average number of all retained orthologues in the three subgenomes was used to estimate the expected retained gene number in each block, and used together with the observed retained gene number, for the gene retention disparity statistics using the χ 2 test. In the GO, IPR (Interproscan) or KEGG enrichment analyses of WGT or tandem genes, the χ 2 test ( N >5) or the Fisher’s exact test ( N ≤5) was used to detect significant differences between the proportion of (WGT or tandem) genes observed in each child GO, IPR or KEGG categories, and the expected overall proportion of (WGT or tandem) genes in the whole genome. Correlation of the gene numbers of WGT-derived paralogous genes with tandem genes in 938 GO terms was tested by Pearson correlation coefficients ( Supplementary Figure 68 ). The Benjamini–Hochberg false discovery rate was performed to adjust the P values [67] . Accession codes: Genome sequence data for B. oleracea have been deposited in the DDBJ/EMBL/GenBank nucleotide core database under the accession code AOIX00000000. Transcriptome sequence data for B. rapa and B. oleracea have been deposited in the DDBJ/EMBL/GenBank Sequence Read Archive (SRA) under the accession codes GSE http://www.ncbi.nlm.nih.gov/nuccore/?term= 43245 and GSE 42891 respectively. How to cite this article: Liu, S. et al . The Brassica oleracea genome reveals the asymmetrical evolution of polyploid genomes. Nat. Commun. 5:3930 doi: 10.1038/ncomms4930 (2014).